Maturation of the proteasome core particle induces an affinity switch that controls regulatory particle association Proteasome assembly is a complex process, requiring 66 subunits distributed over several subcomplexes to associate in a coordinated fashion. Ten proteasome-specific chaperones have been identified that assist in this process. For two of these, the Pba1-Pba2 dimer, it is well established that they only bind immature core particles (CPs) in vivo . In contrast, the regulatory particle (RP) utilizes the same binding surface but only interacts with the mature CP in vivo . It is unclear how these binding events are regulated. Here, we show that Pba1-Pba2 binds tightly to the immature CP, preventing RP binding. Changes in the CP that occur on maturation significantly reduce its affinity for Pba1-Pba2, enabling the RP to displace the chaperone. Mathematical modelling indicates that this ‘affinity switch’ mechanism has likely evolved to improve assembly efficiency by preventing the accumulation of stable, non-productive intermediates. Our work thus provides mechanistic insights into a crucial step in proteasome biogenesis. The selective and timely degradation of polypeptide chains in the cell is important for overall protein homeostasis as well as an integral part of many cellular processes. Many proteins destined for degradation undergo a modification where ubiquitin is covalently attached to lysine residues. The ubiquitin-tag targets substrates to the proteasome, where they are deubiquitinated, unfolded and hydrolysed into short peptide fragments. The proteasome itself is a complex molecular machine containing 66 subunits that must assemble into a 2.5-MDa complex. The subunits are broadly organized into a regulatory particle (RP or 19S, also called PA700 in mammals) that is responsible for substrate recognition, deubiquitination and unfolding, and a proteolytically active core particle (CP or 20S; ref. 1 ). The CP is formed by four stacked rings, each consisting of seven unique α-subunits or seven unique β-subunits, in an α 1–7 β 1–7 β 1–7 α 1–7 arrangement. During CP maturation, the β1 (Pre3), β2 (Pup1) and β5 (Pre2) subunits become proteolytically active through an autocatalytic process that removes propeptides present within these subunits. This occurs when two half CPs, often referred to as 15S or immature CP, dimerize. In yeast, five assembly chaperones, Ump1, Pba1 (also called Poc1), Add66 (also called Pba2 or Poc2), Irc25 (also called Pba3, POC3 or DMP2) and Poc4 (also called Pba4 or Dmp1) have been found to bind the CP before its maturation (reviewed in ref. 2 ). Here, we will refer to these factors as Ump1 and Pba1 to Pba4. Each of these has a human orthologue, known as POMP, and PSMG1 to PSMG4 (also called PAC1 to PAC4). Pba3 and Pba4 form a dimer that binds to α5 (Pup2) and promotes proper α-ring assembly [3] , [4] , [5] . The Pba3-Pba4 dimer must dissociate before the β4 (Pre1) subunit can join the complex owing to extensive steric clashes with this subunit [4] . The chaperone Ump1 associates with immature CP after the α-ring forms. On dimerization of half CPs, Ump1 is retained inside the CP and is degraded as part of the maturation process [6] . Pba1 and Pba2 form a dimer that, similar to Ump1, is present on the half CP, but binds on the outside of the CP cylinder base [7] , [8] . Although Pba1-Pba2 has been shown to prevent α-ring dimerization in mammals [9] , its cellular functions remain poorly characterized. While the CP can be found in the cell by itself (a.k.a. the free CP), in most cases, it acts in consortium with a set of associated factors [10] , [11] . In yeast the RP, Blm10 and Pba1-Pba2 can all bind to the ends of the CP cylinder, although the later has only been shown to bind mature CP in vitro [8] , [12] , [13] , [14] . Blm10 (PSME4/PA200 in humans) has been proposed to function in CP maturation [15] , [16] , CP localization [17] and activation of protein degradation [18] , [19] , [20] . In recent years, it has become clear that these interaction partners all utilize a similar mechanism where carboxy (C)-terminal tails dock into pockets located at the interface between CP α-subunits, often facilitated by a conserved C-terminal HbYX-motif [8] , [12] , [19] , [21] , [22] , [23] , [24] . The C-terminal tail of Pba1 docks into the α5-α6 (Pup2-Pre5) pocket and the Pba2 tail in the α6-α7 (Pre5-Pre10) pocket [8] . Interestingly, the α5-α6 pocket is also utilized by Blm10 and the RP subunits Rpt1 and Rpt5, while the α6-α7 pocket can associate with Rpt4 and Rpt5 (refs 12 , 13 , 14 , 24 ). This suggests that the RP, Blm10 and Pba1-Pba2 compete with one another for CP binding. Since the full α-ring forms early in assembly, one would expect a priori that any CP-binding partner would interact with both mature and immature CPs. While Blm10 can indeed associate with both forms of the CP, the RP is only found associated with mature particles, and Pba1-Pba2 only binds immature CP in vivo [9] , [16] , [25] , [26] , [27] . These observations imply that the binding of these factors to the CP is tightly regulated. The RP chaperones Nas2, Nas6, Hsm3 and Rpn14 (known in humans as PSMD9/p27, PSMD10/gankyrin, PSMD5/S5b and PAAF1/Rpn14, respectively) are one example of this regulation: they all have the capacity to interfere with the association of immature RP subcomplexes and the CP [28] , [29] , [30] , [31] , [32] , [33] , [34] . Despite intense research over the last decade, however, surprisingly little is known about the mechanisms that control the interaction between the CP and its binding partners. In this work, we demonstrate that the Pba1-Pba2 dimer associates tightly with immature CP and prevents them from associating with the RP. Upon CP maturation, however, the affinity of Pba1-Pba2 for the CP changes markedly, presumably owing to a subtle conformational change in the α-ring that impacts the Pba1-Pba2-binding surface. Consistent with this, we observed that the Pba2 tail, which plays a negligible role in mature CP binding, contributes substantially to immature CP binding. Mathematical models of proteasome assembly demonstrated that this ‘affinity switch’ is crucial for achieving high yields of functional molecules. Finally, our results reveal that Pba1-Pba2 is also required for efficient incorporation of α5 and α6 into the immature CP. The Pba1 and Pba2 complex prevents RP binding As mentioned above, Pba1-Pba2 and Blm10 likely compete with each other for binding to the CP α-ring. Consistent with this idea, on purification of proteasomes from pba1 Δ, pba2 Δ or pba1 Δ pba2 Δ yeast strains, we observed increased levels of Blm10 ( Fig. 1a,b and Supplementary Fig. 1a ). However, in vivo Pba1-Pba2 is normally only found on the immature CP, and it has been postulated that one function of Pba1-Pba2 could be to prevent RP from binding to immature CP [8] , [9] , [35] , [36] . To test this hypothesis, we first affinity purified immature CP using TAP-tagged Ump1 ( Fig. 1c,d ). 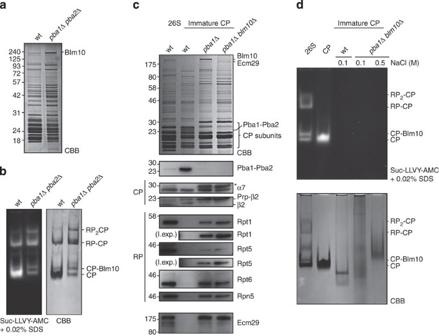Figure 1: Pba1-Pba2 prevents RP association with immature CP. (a) Proteasomes were purified from indicated strains, resolved by SDS–PAGE, and stained with Coomassie brilliant blue (CBB). (b) Native gel analysis of samples fromastained in gel with the proteasome substrate suc-LLVY-AMC (left) or stained with CBB. (c) 26S proteasome or immature CP were affinity purified using ProA-tagged β4 or TAP-tagged Ump1, respectively. Purified complexes were resolved on SDS–PAGE and were stained with CBB (top) or immunoblotted for Pba1-Pba2, indicated proteasome subunits (CP and RP indicate core and regulatory particle subunits, respectively), and Ecm29. The asterisk marks a non-specific band. (d) 26S proteasome and CP were purified using standard protocols. Immature CP was purified and washed with buffers containing the indicated NaCl concentrations. Samples were resolved on a native gel and stained with either suc-LLVY-AMC (top) or with CBB (bottom). wt, wild type. Mass spectrometry analyses confirmed that these purifications contained all seven α-subunits in addition to β1–5, Pba1, Pba2 and Ump1 ( Supplementary Table 1 ). β6 (Pre7) and β7 (Pre4) were undetectable, as has been observed before [37] . The presence of Pba1-Pba2 was also confirmed by immunoblotting ( Fig. 1c and Supplementary Fig. 1b ). Propeptides for β1, β2 and β5 were detected by immunoblotting or mass spectrometry ( Fig. 1c and Supplementary Table 1 ). Taken together, these data indicate that we purified a form of CP that has not matured yet. Figure 1: Pba1-Pba2 prevents RP association with immature CP. ( a ) Proteasomes were purified from indicated strains, resolved by SDS–PAGE, and stained with Coomassie brilliant blue (CBB). ( b ) Native gel analysis of samples from a stained in gel with the proteasome substrate suc-LLVY-AMC (left) or stained with CBB. ( c ) 26S proteasome or immature CP were affinity purified using ProA-tagged β4 or TAP-tagged Ump1, respectively. Purified complexes were resolved on SDS–PAGE and were stained with CBB (top) or immunoblotted for Pba1-Pba2, indicated proteasome subunits (CP and RP indicate core and regulatory particle subunits, respectively), and Ecm29. The asterisk marks a non-specific band. ( d ) 26S proteasome and CP were purified using standard protocols. Immature CP was purified and washed with buffers containing the indicated NaCl concentrations. Samples were resolved on a native gel and stained with either suc-LLVY-AMC (top) or with CBB (bottom). wt, wild type. Full size image RP was not detected above background levels in purifications of immature CP when assessed using several RP-specific antibodies ( Fig. 1c ). To understand how the presence of Pba1-Pba2 might impact interactions of RP with the immature CP, we deleted PBA1 . The deletion of PBA1 resulted in the absence of both Pba1 and Pba2 from immature CP, and the appearance of the RP ( Fig. 1c ). Thus, on deletion of Pba1, the surface of the α-ring becomes available for interaction with RP. Particularly striking was the presence of Ecm29 in this deletion background; Ecm29 is a proteasome-associated protein that only associates with RP-CP species and not free RP or free CP [38] , [39] . It has been found recruited to mutant proteasome forms [29] , [40] , potentially indicating specific recruitment on these samples where RP associates prematurely with CP. Previously, it has been shown that Blm10 associates with both mature CP [17] , [26] , [27] , [38] and immature CP [15] , [16] , [26] . We consistently observed higher levels of Blm10 on immature CP purified from a pba1 Δ strain compared with wild type ( Fig. 1c and Supplementary Fig. 1c ). The deletion of BLM10 together with PBA1 caused a modest further increase of RP binding to immature CP, consistent with the fact that the RP and Blm10 compete for CP binding. Interestingly, a deletion of BLM10 in strains that contain functional Pba1-Pba2 did not cause the RP to associate with immature CP ( Supplementary Fig. 1c ), suggesting that it is mainly the Pba1-Pba2 dimer that blocks association of RP with immature CP. Analysis of immature CP on native gel shows a distinct band that migrates faster than CP and lacks hydrolytic activity ( Fig. 1d ). The deletion of PBA1 resulted in a smear instead of a well-resolved species ( Fig. 1d , lower panel). This smearing is likely caused by different factors associated with the immature CP in the absence of Pba1-Pba2, as including a washing step with high salt resulted in a more distinct band on native gel ( Fig. 1d , lower panel). The band does not migrate similar to wild-type immature CP, which might be caused by the absence of Pba1-Pba2 or a different composition of the immature CP ( Fig. 1c and below). Our results thus indicate that the Pba1-Pba2 dimer shields the immature CP from other factors that can interact with the α-ring surface. RP readily displaces Pba1 and Pba2 from mature CP Crystal structures of Blm10 or Pba1-Pba2 bound to the CP and cryoEM structures of RP-CP complexes show that they bind with the CP exclusively through the α-ring [8] , [12] , [13] , [14] . Since both Ump1-bound immature CP ( Supplementary Table 1 ) and mature CP have a complete α 1–7 ring, it is unclear what drives the difference in binding behaviour observed between mature CP and immature CP. An attractive mechanism that has been proposed posits that Pba1-Pba2 binds to immature CP, but on maturation, Pba1-Pba2 is degraded, which enables the formation of RP-CP complexes. This model is supported by the observation that, on overexpression of a flag-tagged version of the human orthologues PSMG1 (PAC1) or PSMG2 (PAC2), the flag-tagged protein is unstable in HeLa cells [9] . On the other hand, for the yeast orthologues no detectable degradation of Pba1-Pba2 by the mature CP has been observed in vitro [7] , [8] . To test the stability of Pba1-Pba2 in vivo , we conducted chase experiments using an antibody that recognizes endogenous Pba1-Pba2 ( Fig. 2a ). These data suggested that the Pba1-Pba2 dimer is stable. To address the possibility that one of the two subunits is unstable, we next determined steady-state levels of Pba1 and Pba2 in the pba2 Δ and pba1 Δ strains, respectively. Here, a subtle difference in migration between the two proteins can be observed, indicating the antibody recognizes both endogenous Pba1 and endogenous Pba2 ( Fig. 2b ). The strongly reduced signal on deletion of PBA1 or PBA2 might indicate that subunits incapable of forming dimers are subject to degradation in a process unrelated to CP maturation. This finding could potentially explain perceived differences between the yeast and mammalian systems [9] . Finally, we also reintroduced a His-Myc-tagged version of Pba2 in a pba2 Δ background using a CEN plasmid and the endogenous promoter to prevent overexpression. Chase experiments with the later strain also showed both subunits are stable ( Fig. 2c ). In sum, our findings indicate that Pba1-Pba2 is not degraded as part of the CP maturation process in yeast. 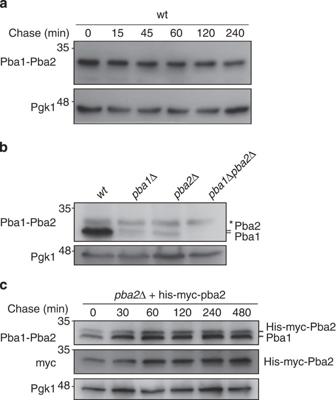Figure 2: Pba1 and Pba2 are stable. (a) Cyclohexamide chase of wild type using antibodies that recognize endogenous Pba1-Pba2. An amount of 100 μg ml−1of cyclohexamide was added to logarithmically growing samples att=0. Samples were collected at indicated times and lysed in SDS sample buffer. Immunoblots show levels of Pba1-Pba2 with Pgk1 as a loading control. Pba1-Pba2 has a long half-life inconsistent with the previously proposed model that Pba1-Pba2 is degraded during the assembly process. (b) Steady-state levels of Pba1-Pba2 in total lysate. (c) Cyclohexamide chase as inabut from a strain that expresses His-Myc-tagged Pba1 from a CEN plasmid under its own promoter. wt, wild type. Figure 2: Pba1 and Pba2 are stable. ( a ) Cyclohexamide chase of wild type using antibodies that recognize endogenous Pba1-Pba2. An amount of 100 μg ml −1 of cyclohexamide was added to logarithmically growing samples at t =0. Samples were collected at indicated times and lysed in SDS sample buffer. Immunoblots show levels of Pba1-Pba2 with Pgk1 as a loading control. Pba1-Pba2 has a long half-life inconsistent with the previously proposed model that Pba1-Pba2 is degraded during the assembly process. ( b ) Steady-state levels of Pba1-Pba2 in total lysate. ( c ) Cyclohexamide chase as in a but from a strain that expresses His-Myc-tagged Pba1 from a CEN plasmid under its own promoter. wt, wild type. Full size image Since CP does not degrade Pba1-Pba2, RP must be able to displace it directly or with the help of other factors. Previous work using surface plasmon resonance had shown that the interaction between mature CP and Pba1-Pba2 is salt labile [8] . We also observe that this interaction can be disrupted with low-salt concentrations when we reconstituted Escherichia coli purified Pba1-Pba2 onto resin-bound CP purified from yeast ( Fig. 3a ). Using biolayer interferometry, we measured a K D of ~1 μM for Pba1-Pba2 with mature CP in 50 mM NaCl ( Supplementary Fig. 2a ), which is similar to the 3-μM reported by Stadtmueller et al. [8] under physiological salt concentrations. Considering the reported nanomolar range affinities between the RP subunit containing complexes and CP [21] , [30] , these findings suggest that the RP will likely displace Pba1-Pba2 from the mature CP. 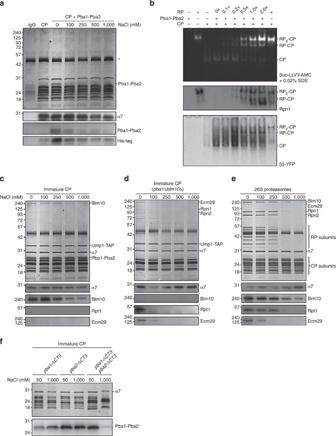Figure 3: CP undergoes affinity switch on maturation. (a) Affinity resin-bound purified CP was reconstituted with heterologously expressed His-tagged Pba1-Pba2 dimer. Samples were washed with buffer containing the indicated NaCl concentrations. Next, samples were resolved on SDS–PAGE and stained with CBB or immunoblotted for the indicated proteins. (b) YFP-tagged CP was first reconstituted with fivefold molar excess of Pba1-Pba2 and challenged with different amounts of purified RP (molar excess over CP indicated). Samples were resolved on a native gel to determine complex composition in samples: Top panel: proteolytic active complexes were visualized using in-gel suc-LLVY-AMC hydrolytic activity assay. Middle panel: native gel was immunoblotted for the RP subunit Rpn1. Lower panel: native gel was analysed for YFP signal. (c–f) Immature CP or 26S proteasome from wild-type or indicated strains were purified, split into different samples and washed with buffer containing the indicated NaCl concentrations. Samples were resolved on SDS–PAGE and stained with CBB or immunoblotted for indicated proteins. The asterisk indicates an IgG resin-derived band. Figure 3: CP undergoes affinity switch on maturation. ( a ) Affinity resin-bound purified CP was reconstituted with heterologously expressed His-tagged Pba1-Pba2 dimer. Samples were washed with buffer containing the indicated NaCl concentrations. Next, samples were resolved on SDS–PAGE and stained with CBB or immunoblotted for the indicated proteins. ( b ) YFP-tagged CP was first reconstituted with fivefold molar excess of Pba1-Pba2 and challenged with different amounts of purified RP (molar excess over CP indicated). Samples were resolved on a native gel to determine complex composition in samples: Top panel: proteolytic active complexes were visualized using in-gel suc-LLVY-AMC hydrolytic activity assay. Middle panel: native gel was immunoblotted for the RP subunit Rpn1. Lower panel: native gel was analysed for YFP signal. ( c – f ) Immature CP or 26S proteasome from wild-type or indicated strains were purified, split into different samples and washed with buffer containing the indicated NaCl concentrations. Samples were resolved on SDS–PAGE and stained with CBB or immunoblotted for indicated proteins. The asterisk indicates an IgG resin-derived band. Full size image To further test this, we developed an in vitro reconstitution assay. First, we combined mature CP with increasing ratios of Pba1-Pba2 to determine the stoichiometry of binding on native gel. Pba1-Pba2 binds to the CP but does not cause a mobility shift ( Supplementary Fig. 2b ). Since a fivefold excess of Pba1-Pba2 showed maximum CP binding, we challenged reconstitutions with that ratio of Pba1-Pba2 to CP with increasing amounts of RP ( Fig. 3b ). We found that the RP associates with the CP starting at low concentrations where Pba1-Pba2 is in 20-fold excess over RP. This indicates that the RP can readily replace Pba1-Pba2 bound to mature CP. These analyses are complicated by a small amount of active RP 2 -CP that co-purifies with our RP preparations (ref. 38 and Fig. 3b , lane 2). However, looking at the singly capped RP-CP or visualizing exclusively the reconstituted CP by utilizing YFP-tagged CP ( Fig. 3b , lowest panel), we know that the RP is reconstituted onto Pba1-Pba2-CP complexes. These data suggest that Pba1-Pba2 bound to mature CP cannot prevent RP association. Hence, there is no need for Pba1-Pba2 degradation to produce RP-CP complexes. A switch in affinity on CP maturation We hypothesized that a specific mechanism must exist that ensures Pba1-Pba2 cannot be replaced by RP when bound to immature CP. This could involve regulatory proteins, similar to the RP chaperones that associate with RP complexes. However, those chaperones cannot fully prevent RP-immature CP association as we observed RP binding in pba1 Δ cells ( Fig. 1c ). As an alternative mechanism, we envisioned a conformational change in the α-ring on maturation that changes the binding surface between the CP and associated proteins. In general, the CP has more structural plasticity then has been appreciated [41] . More specifically, during the final steps of CP maturation, β7 is incorporated, immature CP dimerizes, autoproteolytic cleavage activates the three active sites (β1, β2 and β5) and Ump1 is degraded [2] . The β7 subunit is in direct contact with the α-subunits that bind to Pba1-Pba2, α6 and α7 (ref. 8 ), thereby providing a direct opportunity to induce a conformational change in the α-ring. Alternatively, autoproteolytic activation might provide a trigger that induces a conformational change in CP, as modification of active sites has been shown to change properties of the α-ring [38] , [42] . To test for differences in binding behaviour between mature and immature CP, we characterized the salt dependence of several different interactions. First, we used TAP-tagged Ump1 to purify immature CP associated with endogenous Pba1-Pba2. Here, even washes with buffers containing 1 M NaCl washed off very little of the Pba1-Pba2 complex from immature CP ( Fig. 3c ). This is in sharp contrast to the Pba1-Pba2 association with mature CP, which is highly salt labile ( Fig. 3a and ref. 8 ). Next, to test whether the RP also shows a change in binding behaviour, we purified immature CP from the pba1 Δ blm10 Δ strain and exposed it to washes with different salt concentrations. In these samples, the RP consistently washes off in buffers containing 100 mM NaCl ( Fig. 3d ), while 250–500 mM NaCl is required to disrupt the binding between RP and mature CP ( Fig. 3e and ref. 39 ). These data suggest that the immature CP has a high affinity for Pba1-Pba2 and a low affinity for the RP. On maturation, the affinities are reversed and the RP has a much higher affinity for the mature CP than Pba1-Pba2. For RP binding to the immature CP, we cannot exclude that the reduced binding is due to differences in immature CP composition on PBA1 deletion (see below). However, in reconstitution assays, we were unable to expel Pba1-Pba2 from normal immature CP, even though the base subcomplex of the RP efficiently reconstituted on mature CP ( Supplementary Fig. 2c,d ) and can expel Pba1-Pba2 from mature CP ( Fig. 3b ). Interestingly, the binding of Blm10 to both mature and immature CP shows a disruption of the interaction at similar salt concentrations, suggesting that Blm10 is not sensitive to the affinity switch (compare Fig. 3c,e ). This is consistent with the fact that Blm10 has been observed on mature as well as immature CP under physiological conditions [17] , [26] . In all, these data reveal an affinity switch during CP maturation that at least in part can explain the exclusive binding of Pba1-Pba2 to immature CP and RP to mature CP. The Pba2 tail contributes to the affinity switch Pba1 and Pba2 both contain an HbYX-motif that is required for functionality [7] , [8] , and a crystal structure of Pba1-Pba2 bound to the CP shows that both C termini dock in a specific α-pocket [8] . Interestingly, in the interaction with the mature CP, the tail of Pba2 contributes only minimally to binding, since its deletion reduces the affinity with only two- to three-fold [8] . In comparison, deleting the tail of Pba1 reduced the affinity >100-fold. The differential contribution to the affinity can be rationalized through analysis of the structure itself. Pba2 binds in an unusual manner to the CP, lacking several hydrogen bonds commonly observed for HbYX-motif binding in the α-pockets (for example, for the HbYX of Pba1 or Blm10). For example, the hydroxyl group of the tyrosine residue in the Pba2 HbYX-motif is far (4.2 Å) removed from the closest potential hydrogen bond partner [8] , [12] . Despite the apparent minor role in binding to the CP, the HbYX-motif of Pba2 is physiologically relevant, since mutant strains with a truncated tail show phenotypes similar to mutants lacking the Pba1 HbYX-motif [7] , [8] . Only after deletion of both HbYX-motifs, however, do strains show phenotypes that mimic pba 1Δ strains [7] , [8] . Hence, the HbYX-motif of Pba2 has an unidentified but important physiological function. We hypothesized that the HbYX-motif of Pba2 is more important for binding with the immature CP as compared with the mature CP, thereby contributing to the observed affinity switch. Such a difference might arise from small changes in the conformation of the α6-α7 pocket, or from the fact that changes in Pba1-α5-α6 interactions could limit the ability of Pba2 to interact fully with its pocket in the mature CP. The model described above predicts that both the Pba2 and Pba1 HbYX-motif would have a role in binding to the immature CP. To test this, we deleted the HbYX-motif from Pba1 ( pba1- ΔCT3), Pba2 ( pba2- ΔCT3) or both together ( pba1- ΔCT3 pba2- ΔCT3) in an Ump1-Tap-tagged background. Next, we tested the salt lability of Pba1-Pba2 binding to immature CP. To our surprise, Pba1-Pba2 remained bound to immature CP in both the pba1- ΔCT3 and pba2- ΔCT3 background even after washes with 1 M NaCl ( Fig. 3f ). The binding of Pba1-Pba2 to the immature CP is thus very different compared with the mature CP, as the latter showed a highly salt-dependent interaction that depends largely on the Pba1 tail ( Fig. 3a and ref. 8 ). Only after deletion of both the Pba1 and Pba2 HbYX-motif ( pba1- ΔCT3 pba2- ΔCT3) did we observe loss of binding of the Pba1-Pba2 complex to immature CP with high-salt washes ( Fig. 3f ). Thus, in contrast to binding to mature CP, both the Pba1 and Pba2 HbYX-motif contribute substantially to the affinity of Pba1-Pba2 for immature CP. This suggests that a major contributor to the molecular mechanism of the affinity switch derives from differences in how the Pba2 HbYX-motif docks into the α6-α7 pocket. Pba1 and Pba2 contribute to α5 and α6 incorporation On purification of immature CP from a pba1 Δ strain, we noticed a reduced level of a specific proteasome CP subunit after SDS–PAGE analysis (compare Fig. 3c,d ). Based on the running behaviour, previous assignments by other laboratories [26] , [43] and our own mass spectrometry analysis ( Fig. 4a,b and Table 1 ), we determined this was the subunit α6. This suggests that there is a reduced level of α6 present in immature proteasomes in the absence of Pba1. Additional mass spectrometry analysis suggested that besides α6 there might also be reduced levels of α5. To test this, we ran two-dimensional (2D) gels of mature CP from wild type and immature CP from wild-type and pba1 Δ strains ( Fig. 4c and Supplementary Fig. 3 ). These gels confirmed the substantial reduction in levels of α5 and α6 from immature CP purified from pba1 Δ strains. Pba1 thus likely has a role in efficient incorporation of α5 and α6, similar to Pba3-Pba4, which has a role in controlling α3 (Pre9) and α4 (Pre6) incorporation. However, α5 and α6 are essential subunits of the proteasome, making a potential role for Pba1-Pba2 in formation of alternative proteasomes, as was proposed for Pba3-Pba4 (ref. 3 ), unlikely. Considering the thermodynamic stability of rings once they have formed [44] , [45] , [46] , the reduced level of these two subunits most likely indicates a slow incorporation of these subunits into the α-ring in a pba1 Δ strain. However, an alternative or additional role of Pba1-Pba2 might be the stabilization of α5 and α6 once they have been incorporated into the α-ring, in particular, since α5 and α6 appear to be absent in the high-salt wash of the pba1- ΔCT3 pba2- ΔCT3 strain ( Fig. 3f ). 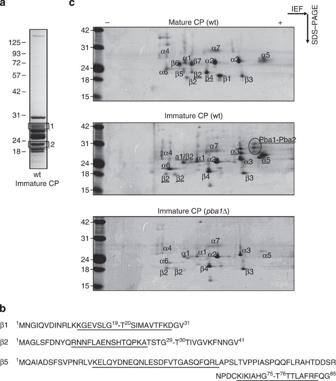Figure 4: Pba1-Pba2 are required for efficient incorporation of α5 and α6. (a) Immature CP from wild-type strain was purified and resolved on SDS–PAGE. Two bands that were consistently absent or reduced in apba1Δ background (Figs 1cand3c,d) were excised and submitted to mass spectrometry analysis for identification (Table 1). Band 1 was identified as Pba1 and Pba2, while α6 was the major component of band 2, consistent with previous assignments15,26,43. (b) Unique peptides from the mass spectrometry analyses inathat cover regions of the propeptides of β1, β2 and β5 are underlined with the pro-peptide sequence in bold. (c) Purified mature or immature CP from indicated strains were resolved by 2D gel electrophoresis using a non-linear ZOOM IPG strip (pH 3–10) followed by SDS–PAGE. Gels were stained with CBB. Proteins spots were assigned based on immunoblotting (Supplementary Fig. 3a), mass spectrometry analyses (underlined andSupplementary Fig. 3b) and previous assignments26,43. wt, wild type. Figure 4: Pba1-Pba2 are required for efficient incorporation of α5 and α6. ( a ) Immature CP from wild-type strain was purified and resolved on SDS–PAGE. Two bands that were consistently absent or reduced in a pba1 Δ background ( Figs 1c and 3c,d ) were excised and submitted to mass spectrometry analysis for identification ( Table 1 ). Band 1 was identified as Pba1 and Pba2, while α6 was the major component of band 2, consistent with previous assignments [15] , [26] , [43] . ( b ) Unique peptides from the mass spectrometry analyses in a that cover regions of the propeptides of β1, β2 and β5 are underlined with the pro-peptide sequence in bold. ( c ) Purified mature or immature CP from indicated strains were resolved by 2D gel electrophoresis using a non-linear ZOOM IPG strip (pH 3–10) followed by SDS–PAGE. Gels were stained with CBB. Proteins spots were assigned based on immunoblotting ( Supplementary Fig. 3a ), mass spectrometry analyses (underlined and Supplementary Fig. 3b ) and previous assignments [26] , [43] . wt, wild type. Full size image Table 1 Mass spectrometry analyses of band 1 and band 2 in Fig. 4a . Full size table Preventing premature RP binding improves assembly efficiency Our data provide experimental evidence and mechanistic insight into a role of Pba1-Pba2 in preventing binding of RP to immature CP. To better understand the importance of the observed affinity switch, we developed a mathematical model in which we manipulated the affinity of Pba1-Pba2 for the CP α-ring. In our model of proteasome assembly, the α-ring is nucleated by the formation of an α5-α6 dimer, and we kept the roles of the Pba3-Pba4 chaperone [1] , [47] , [48] implicit. After α-dimers form, other α-subunits can bind on either end of the complex, eventually leading to the formation of the α-ring. We ignored subsequent steps in CP maturation (addition of the β-subunits, half proteasome dimerization and so on) in order to reduce the complexity of the model. To test the effect of the proposed affinity switch, we used various affinities for Pba1-Pba2 dimer bound to intermediates as well as the full α-ring. We only included fully formed RPs in this model, assuming that the RP chaperones would prevent association between immature RPs and CP subunits [28] , [29] , [30] , [31] , [33] , [34] . Finally, since the Rpt ring of the RP makes many contacts with the α-subunits of the CP [13] , [49] , RP binding to α-ring structures was considered to be stable when the α-intermediate in question contained >1 subunit [44] , [45] , [46] . We used this model to analyse how proteasome assembly efficiency (defined as the formation of fully active 26S RP-CP complexes) depends on the concentration of Pba1-Pba2 for three different scenarios. In the first, we implemented the affinity switch that was implied by our data ( Fig. 5a,b , black lines). In the affinity switch model, the K D of Pba1-Pba2 for the mature CP was taken to be 1 μM ( Supplementary Fig. 2a ), and the K D of Pba1-Pba2 for immature CP was taken to be three orders of magnitude stronger (1 nM) to represent the lack of dissociation of the chaperones from immature CP even in high salt ( Fig. 3c ). The other two scenarios lacked an affinity switch, and the affinity of Pba1-Pba2 for mature and immature CP was either low (1 μM, ‘low affinity’; Fig. 5a,b , red lines) or high (1 nM, ‘high affinity’; Fig. 5a,b , green lines). 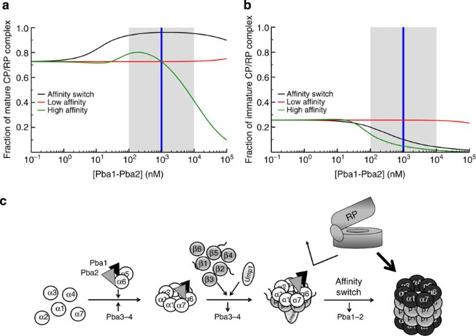Figure 5: Pba1-Pba2 prevents assembly deadlock. (a) Mathematical models were designed to investigate the function of Pba1-Pba2 (see text for details). The graph explores three scenarios. In the first (black line), we incorporated an affinity switch in our model. Theyaxis shows fraction of assembled proteasomes, which reaches 1 within the likely physiological range of concentrations of Pba1-Pba2 in the presence of an affinity switch (grey area). The second scenario (green line) assumed a high affinity rather than an affinity switch, whereas the third considered a low affinity (red line). (b) This graph displays the fraction of complexes in which the RP is associated with the CP before CP maturation, thereby yielding unproductive, deadlocked complexes. (c) Proposed conceptual model for the role of Pba1-Pba2 in CP maturation (see text for details). Figure 5: Pba1-Pba2 prevents assembly deadlock. ( a ) Mathematical models were designed to investigate the function of Pba1-Pba2 (see text for details). The graph explores three scenarios. In the first (black line), we incorporated an affinity switch in our model. The y axis shows fraction of assembled proteasomes, which reaches 1 within the likely physiological range of concentrations of Pba1-Pba2 in the presence of an affinity switch (grey area). The second scenario (green line) assumed a high affinity rather than an affinity switch, whereas the third considered a low affinity (red line). ( b ) This graph displays the fraction of complexes in which the RP is associated with the CP before CP maturation, thereby yielding unproductive, deadlocked complexes. ( c ) Proposed conceptual model for the role of Pba1-Pba2 in CP maturation (see text for details). Full size image As can be seen in Fig. 5a , the behaviour of these three scenarios is quite different. The presence of an affinity switch results in very high assembly yield compared with the absence (that is, very low concentrations) of Pba1-Pba2; going from 75% to almost 100%. The improved assembly results from a decrease in RP binding to immature CP intermediates ( Fig. 5b ). When the concentration of Pba1-Pba2 reaches unphysiologically high levels (~100 μM), it overcomes the affinity switch and begins to interfere with 26S assembly by blocking RP association with mature CP ( Fig. 5a ). The 75% yield in the absence of Pba1 or Pba2 fits well with in vivo data, where the deletion of Pba1 or Pba2 does not cause a severe phenotype [25] , [26] , but likely causes a reduction in assembly yield substantial enough to explain synergistic phenotypes with other proteasome mutants [25] , [26] . If we remove the affinity switch, however, the robust increase in assembly yields owing to the presence of Pba1-Pba2 is no longer observed in the model. When affinities are uniformly low ( Fig. 5a , red line), Pba1-Pba2 simply does not bind either immature or mature CP well enough at physiological concentrations to have an impact on assembly yields. When affinities are uniformly high, on the other hand, Pba1-Pba2 blocks RP binding to both the mature and immature CP, thereby resulting in lower yields ( Fig. 5b , green line). While the results in Fig. 5 suppose a particular concentration of both RP and CP subunits in the cell, independent variations in these concentrations do not influence the overall trends observed in the model ( Supplementary Fig. 4a ). Similarly, changes to the size of the affinity switch also do not influence the general behaviour of the model ( Supplementary Fig. 4b ). Our model thus provides a robust explanation for the functional role of the Pba1-Pba2 affinity switch; by blocking premature RP-CP association, these chaperones prevent the stabilization of intermediates that would lead to CP assembly deadlock [44] . The switch from a high-affinity to low-affinity binding conformation on CP maturation ensures that the chaperone ‘gets off’ the complex at the right time, thereby allowing the RP to bind once the CP is fully formed. Fig. 5c summarizes our current conceptual model of the role of Pba1-Pba2. CP assembly starts with the formation of the α 1–7 ring. In the early steps of assembly, both the Pba1-Pba2 and the Pba3-Pba4 dimers have a role in efficient ring formation. Pba3-Pba4 has a role in ring nucleation and ensures incorporation of α3(ref. 3 ). The presence of Pba1-Pba2 ensures the efficient incorporation or stabilization of α5 and α6. Next, the β-subunits assemble onto the α ring; at this step in the process, Pba3-Pba4 must dissociate from the complex to avoid steric clashes with the β4 subunit [4] . However, Pba1-Pba2 remains bound until late in the assembly process, shielding the external surface of the α-ring from RP and Blm10 and also preventing α-ring dimerization [9] . After assembly of the β-ring, several steps must occur including dimerization of immature half proteasomes and autocatalytic activation [1] , [48] . Our results show that maturation of the CP causes a change in the binding of Pba1-Pba2 to the CP. While the structural basis of the affinity switch has yet to be determined, our data suggest that conformational changes in the CP that accompany maturation impact the capacity of the HbYX-motif on Pba2 to interact with the α6-α7 pocket. The affinity switch we have identified allows the chaperone to specifically protect the immature CP from interactions with regulatory factors, thereby preventing the formation of unproductive complexes that decrease the assembly yield of functional proteasomes. It is likely that other assembly chaperones (particularly those that bind to immature RPs, for example, Nas6) utilize a similar mechanism, preventing association with larger assemblies before completion of subcomplex assembly. Small structural changes that accompany maturation likely reduce the affinity for these chaperones, allowing for the coordinated exchange of possible binding partners during the assembly process. Yeast techniques and reagents Yeast strains used are summarized in Supplementary Table 2 . Genomic manipulation of yeast was done using a PCR-based approach [50] , [51] . On transformation of yeast, successful integration was confirmed by positive PCR for integration and negative PCR for wild type. Pba1 knockout primer pRL 252 (5′-AAGATATCATCGCACTACAGTAAAATTTTCATTTATAGCGCGGATCCCCGGGTTAATTAA-3′) and pRL253 (5′-CTCTTTCACTCGCCATTACTGACATTCTGTGATCGCCATCATCGATGAATTCGAGCTCGT-3′) and Pba2 knockout primers pRL254 (5′-ACTTCAGGAAAGAATAGCACAAAACCCAAAGGAACATACGCGGATCCCCGGGTTAATTAA-3′) and pRL255 (5′-TATATGCACTTGTATAGAAAACAGATATACTTCTCGGTTCATCGATGAATTCGAGCTCGT-3′) were used together with templates pAG25 (natMX4) and pAG32 (hphMX4; ref. 51 ) in a PCR to prepare DNA for yeast transformation. To create a strain deleted for Blm10, genomic DNA from a blm10Δ strain [27] was used as template for PCR with the following primers: pf2Blm10 (5′-CTGTCATCAGGGCTTG-3′) and pr2Blm10 (5′-GTTGATCATTCTCAGTGG-3′). To produce C-terminal truncation of Pba1 that deleted the codons coding for the last three amino acids of Pba1, pba1- ΔCT3, primers pRL210 (5′-TGGAGGTGTGATAGCGCGGCAATTGGTGCACAATCAGGCTGAGGCGCGCCACTTCT-3′) and pRL253 (5′-CTCTTTCACTCGCCATTACTGACATTCTGTGATCGCCATCATCGATGAATTCGAGCTCGT-3′) were used with pFA6a-3HA-kanMX6 as template [50] . To create pba2- ΔCT3 primers pRL211 (5′-GCATACGGAATGGCGGATGCAAGAGATAAATTTGTAGATTGAGGCGCGCCACTT-3′) and pRL255 (5′-TATATGCACTTGTATAGAAAACAGATATACTTCTCGGTTCATCGATGAATTCGAGCTCGT-3′) were used with pFA6a-3HA-TRP1 as template [50] . Integrations were confirmed by PCR and sequencing. To create a strain with C-terminal YFP tag fused to β2, we used a knock-in DNA fragment synthesized from pDH6 as template (a generous gift of the Yeast Resource Center) in a PCR with primers pRL73 (5′-AATATTTGTGACATACAAGAAGAACAAGTCGATATAACGGCTGGTCGACGGATCCCCGGG-3′) and pRL74 (5′-TGATTTACTATACTAAAATATACTTAAGTTCTATGTTTTACTATCGATGAATTCGAGCTCG-3′). Gibson cloning kit (NEB) was used to create a CEN plasmid that expresses His-Myc Pba2 utilizing the promoter and terminator of PBA2 . pRS416 was digested with BamHI and mixed with two PCR products that were generated using yeast genomic DNA as template together with the following primer pairs: pRL274 (5′-TGCAGCCCGGGGGAGTCCTCGATTTGACTGGAAAC-3′) with pRL275 (5′-CAGATCTTCCTCGCTAATCAGCTTCTGCTCCATCGTATGTTCCTTTGGGTTTTGTGC-3′) and pRL276 (5′-GAGGAAGATCTGCACCACCATCACCATCACCATGGAAGCAGCTGCCTGGTGTTGCC-3′) with pRL277 (5′-CGCTCTAGAACTAGTGAAATTCAAAGAGATGTTACAGAC-3′) using the manufacturer’s protocol. The resulting plasmid is pCEN-His-Myc-Pba2 (pJR643). A polyclonal antibody that recognizes the Pba1-Pba2 complex was generated using a standard immunization protocol (Rockland Immunochemicals, Inc.) with a dimer of Pba1 and His-tagged Pba2 purified from E. coli as the antigen ( Supplementary Fig. 2b ). Ecm29 and Rpn5 were detected using polyclonal antibodies kindly provided by Dr Dan Finley (Harvard Medical School, Boston, MA). Monoclonal antibodies for α7 and Rpt5 were kindly provided by Dr William Tansey (Vanderbilt-Ingram Cancer Center, Nashville, TN). Polyclonal anti-pup1 (β2) antibody was a generous gift from Dr R. Jürgen Dohmen (University of Cologne, Cologne, Germany). Antibodies recognizing Rpt1 and Blm10 were purchased from ENZO Life Sciences and THE HIS-tag antibody was obtained from GenScript. Peroxidase-conjugated secondary antibodies were purchased from Jackson ImmunoResearch Laboratories, and for Fig. 2f Rabbit TrueBlot IgG HRP from Rockland Immunochemicals was used. Anti-Myc antibody (9E10) was derived from an ATCC hybridoma cell line (no. CRL1729). The monoclonal anti-pgk-1 antibody was purchased from Life Technologies (no. 459250). All antibodies were used in 1:1,000 dilutions in Tris Buffered Saline with Tween 20, except those against pgk-1 (1:10,000), Pba1-Pba2 (1:500), Myc (1:5) and Rpt5 (1:5,000). Uncropped images from the most important immunoblots are provided in Supplementary Fig. 5 . Proteasome purification The purification of proteasomes and proteasome subcomplexes from yeast were in essence performed as described previously [29] , [30] , [31] , [38] . Specific yeast strains were grown overnight in 2–3 l of YPD media (final A600 ~10.0). Cells were collected and washed with H 2 O. Pellets were resuspended in 1.5 pellet volume of lysis buffer (50 mM Tris (pH 8.0), 5 mM MgCl 2 , 1 mM EDTA and 1 mM ATP) and lysed by French press (1,200 psi). Lysates were cleared by centrifugation (10,000 g for 30 min) and supernatant was filtered through cheesecloth before incubation with IgG beads (MP Biomedical; 0.75 ml resin bed volume per 25 g of cell pellet). After 1 h of incubation (rotating at 4 °C), IgG beads were collected in an Econo Column (Bio-Rad) and washed with 50-bed volumes of ice-cold wash buffer (50 mM Tris (pH 7.5), 5 mM MgCl 2 , 100 mM NaCl, 1 mM EDTA and 1 mM ATP). Next, material was washed with 15-bed volumes of cleavage buffer (50 mM Tris (pH 7.5), 5 mM MgCl 2 , 1 mM dithiothreitol (DTT) and 1 mM ATP). Bead-bound proteasome complex was either directly analysed by loading on the SDS–PAGE after boiling with equal amount of 2 × SDS–PAGE sample buffer or eluted by incubation with His-Tev protease (Invitrogen). Protease was removed by incubation with Talon resin before concentrating the proteasome complexes using 100 kDa concentrator (Pall Life Sciences). Proteasome purifications were used directly or stored at −80 °C in the presence of 5% glycerol. Reconstitution assay Proteasome CPs and RPs were purified as described previously [38] using strain sJR797 and SY36, respectively. An amount of 12.5 nM of CP and 62.5 nM of purified Pba1-Pba2 dimer protein were reconstituted in reconstitution buffer (50 mM Tris‐HCl (pH 7.5), 5 mM MgCl 2 , 1 mM ATP, 50 mM NaCl and 10% glycerol; Supplementary Fig. 2 ) and incubated for 30 min at 30 °C. Next, increasing amounts of RP were added to different tubes (0, 1.25, 2.5, 6.25, 12.5 and 25 nM in reconstitution buffer), and the volume was adjusted to 20 μl for all samples. Samples were incubated for 30 min at 30 °C. To analyse the reconstitution assay, 1/10 volume of native gel loading buffer (50 mM Tris‐HCl (pH 7.4), 50% glycerol and 60 ng ml −1 xylene cyanol) was added and samples were loaded onto native gel [52] . First, gels were analysed by in-gel protease activity using LLVY-AMC as substrate. Next, samples were transferred to polyvinylidene fluoride membrane for immunoblotting as described previously [38] . Expression and purification of Pba1 and Pba2 complex The ORF of PBA1 was amplified from yeast gDNA by PCR using primers pRL145 (5′-CTGTTGGATCCATGCTTTTTAAACAATGGAATGACTTACCAG-3′) and pRL146 (5′-CGGGAATTCTCATATATATAGGCCTGATTGTG-3′). The PCR product was cloned into pNU247, a pGEX-6PK-1-derived plasmid, using the enzymes BamHI and EcoRI. The ORF of PBA2 was amplified from yeast gDNA by PCR using primers pRL147 (5′-GGCAGATCTTGAAAACCTGTATTTCCAGGGACAGGATCCGATGAGCTGCCTGGTGTTG-3′) and pRL148 (5′-CTCGAGCTCTCAATTGTATAAATCTAC-3′). The PCR product was cloned into pRSF Duet-1 (EMD Millipore) using BglII and BamHI sites. The resulting plasmids were introduced together into Rosetta DE3 cells (Stratagene) to enable co-purification of glutathione S -transferase (GST)-tagged Pba1 and His-tagged Pba2. Transformed cells were inoculated in Luria-Bertani medium supplemented with kanamycin, ampicillin and chloramphenicol, and were incubated at 37 °C with shaking at 200 r.p.m. At an OD 600 of 0.6, isopropyl-β- D -thiogalactoside was added to 0.1 mM final concentration and the culture was incubated overnight at 37 °C with shaking. Cells were harvested by centrifugation (6,000 g , 10 min at 4 °C), washed in sterile H 2 O and resuspended in lysis buffer (20 mM Tris-HCl (pH 8.0), 100 mM NaCl and 0.1% Triton X-100) supplemented with protease inhibitor cocktail tablet (Roche). Lysis was performed at 900 psi using a French press system. Lysate was cleared by centrifugation (10,000 g , 30 min at 4 °C). To the clear cell lysate, glutathione agarose resin (GoldBio; 100 μl per 100 ml culture) was added and samples were incubated at 4 °C for 1 h. The resin was washed four times with total 50-bed volumes of PBS buffer containing 0.1% Triton X-100 and 0.02% Na-azide. To elute the Pba1-Pba2 dimer, resin was washed and resuspended in GST precision cleavage buffer (50 mM Tris-HCl (pH 6.8), 150 mM NaCl, 1 mM DTT and 0.01% Triton X-100) and incubated overnight in the presence of GST precision protease. Eluted material was further purified using an AKTA purifier with a HiLoad Superdex 200 column equilibrated with reconstitution buffer (50 mM Tris-HCl (pH 7.5), 5 mM MgCl 2 , 50 mM NaCl, 1 mM ATP and 1 mM DTT). Fractions containing Pba1-His-Pba2 protein were collected and concentrated using 10 KDa concentrator (Pall Life Sciences). Salt-dependent binding To test for salt-dependent binding as described in Fig. 2 , indicated strains were processed using our standard proteasome purification protocol, up until the IgG beads washing step. Here, 20-bed volumes of a different wash buffer were used (50 mM Tris‐HCl (pH 7.5), 5 mM MgCl 2 , 1 mM EDTA, 1 mM ATP and 0.1% Triton X-100). Next, washed IgG beads were distributed equally among five Eppendorf tubes. Beads were resuspended in five-bed volumes of buffer (50 mM Tris‐HCl (pH 7.5), 5 mM MgCl 2 , 1 mM EDTA, 1 mM ATP and 0.1% Triton X-100) containing different concentrations of NaCl (0, 100, 250, 500 and 1,000 mM) and incubated for 3 min at room temperature under rotation. Beads were pelleted by centrifugation (500 g , 1 min at 4 °C). This washing step was performed for two additional times. Next, beads were washed twice with five-bed volumes of low-salt buffer (50 mM Tris‐HCl (pH 7.5), 5 mM MgCl 2 , 1 mM DTT, 1 mM ATP and 0.1% Triton X-100). Finally, samples were resuspended in 2 × SDS–PAGE sample buffer and loaded on 12% SDS–PAGE. Binding affinity measurements Binding kinetics of the His-tagged Pba1-Pba2 to purified mature CP were measured using biolayer interferometry on a BLItz instrument (ForteBio). The Pba1-Pba2 complex was immobilized on a Ni-NTA biosensor using a 4.5-μM solution. Different concentrations of CP (from 0.0 to 1.8 μM) in reconstitution buffer (50 mM Tris (pH 7.5), 5 mM MgCl 2 , 50 mM NaCl, 1 mM ATP and 10% glycerol) were used as analyte. Advanced kinetic experiment setup was used and kinetic parameters ( k on and k off ), and affinity ( K D ) were calculated from a global fit (1:1) of the BLItz instrument data using the BLItz software. Cyclohexamide chase Specific yeast strains were grown overnight in 5 ml of YPD or minimal selection media. The next day, cells were diluted to OD 600 0.3 in fresh medium and allowed to grow up to logarithmic growth (OD 600 1.0). Cells were then treated with cyclohexamide (100 μg ml −1 ) for the indicated number of minutes, and cells that were equivalent to 1 ml of OD 600 2.0 of cells were collected at each time point. Equal amounts of protein extract from each time point were then loaded on 11% SDS–PAGE and a western blot was performed. 2D gel analysis Ump1-containing immature CP complexes were purified from sJR792 and sJR793 using the proteasome purification protocol described above. An amount of 25 μg of each purified complex was vacuum dried and rehydrated in 140 μl of 2D rehydration buffer (8 M urea, 2% CHAPS, 20 mM DTT, 0.002% bromophenol blue and 0.5% ZOOM carrier ampholytes pH 3–10 (Life Technologies)). Isoelectric focusing was done using ZOOM IPG strips—pH 3-10NL (non-linear) according to the manufacturer’s protocol. Next, IEF strips were incubated in 1 × SDS–PAGE sample buffer for 10 min. Strips were inserted into 12% SDS–PAGE to run for the second dimension. After electrophoresis, gels were either stained with Coomassie brilliant blue or used to transfer samples to polyvinylidene fluoride for subsequent analysis by immunoblotting. Mass spectrometry Mass spectrometry-grade solvents were purchased from Burdick & Jackson or Baker, sequencing grade trypsin from Promega and other solutions were the highest grade available from Sigma-Aldrich. For digestions, samples were denatured by SDS–PAGE (gel bands or spots), reduced with Tris (2-carboxyethyl)phosphine, alkylated with 2-iodoacetamide, and digested overnight with 4 μg ml −1 trypsin, using Tris-HCl (pH 8.5) to buffer all solutions. For liquid chromatography tandem mass spectrometry analyses, samples were analysed on a hybrid LTQ-Orbitrap mass spectrometer (Thermo Fisher Scientific) coupled to a New Objectives PV-550 nanoelectrospray ion source and an Eksigent NanoULC chromatography system. Peptides were analysed by trapping on a 5-cm pre-column using a vented column configuration, followed by analytical separation on a New Objective 75 μm inner diameter fused silica column with an integral fused silica emitter, packed in house with 40 cm of 3-μm Magic C18 AQ beads. Peptides were eluted using a 5–40% acetonitrile/0.1% formic acid gradient performed over 100–200 min at a flow rate of 250 nl min −1 . During elution, samples were analysed using Top Six methodology, consisting of one full-range fourier transform mass spectrometry scan (nominal resolution of 60,000 full-width at half-maximum, 300–2,000 m/z ) and six data-dependent MS/MS scans performed in the linear ion trap. MS/MS settings used a trigger threshold of 8,000 counts, monoisotopic precursor selection, and rejection of specific parent ions. Rejected parent ions had unassigned charge states, were previously identified as contaminants on blank gradient runs, or had been previously selected for MS/MS (dynamic exclusion at 150% of the observed chromatographic peak width). MS data analysis Centroided ion masses were extracted using the extract_msn.exe utility from Bioworks 3.3.1 and were used for database searching with Mascot v2.2.04 (Matrix Science). The search parameters used were as follows: 6.0 p.p.m. parent ion mass tolerance, 0.6 Da fragment ion tolerance, allow up to one missed cleavage; and variable modifications, carbamidomethyl (C), oxidation (M), propionamide (C) and pyro-glu (N-term Q). Database searching was conducted using the Saccharomyces cerevisiae plus filter, resulting 134,809 entries. Peptide and protein identifications were validated using Scaffold v2.2.00 (Proteome Software) and the PeptideProphet algorithm [53] . Searches were performed using thresholds of 1% peptide false discoveries and 1% protein false discoveries with at least two peptides identified. Proteins that contained similar peptides and could not be differentiated based on MS/MS analysis alone were grouped to satisfy the principles of parsimony. MALDI-TOF analyses Protein spots and gel blanks from 2-D gels were excised and digested with trypsin (8 μg ml −1 ). For MALDI-TOF (matrix-assisted laser desorption ionization–time of flight) analyses, peptide extracts were mixed with alpha-cyano-4-hydroxy-cinnamic acid and analysed on a Voyager DE-PRO instrument operated in reflectron mode. Individual TOF spectra were routinely externally calibrated with a known peptide mix (100 p.p.m. accuracy). Supplemental strategies included desalting and concentration of peptide extracts on miniature C-18 affinity columns (OMIX tips from Agilent) and internal recalibration of MALDI-TOF spectra using trypsin autolysis products (20 p.p.m. accuracy). MALDI-TOF ion peaks were extracted using Data Explorer 4.0. Spectra were deisotoped at a peak detection threshold of 5% base peak intensity, and a peak list from the m/z range 500–3,000 was built using the five most intense peaks from each 100- m/z interval. Alternatively, weaker spectra were analysed using manually optimized peak detection windows that visually tracked the baseline noise threshold. Peptide mass fingerprint searches were conducted using MASCOT (v2.2). Protein identifications were accepted if their MASCOT probability-based MOWSE scores (PBM) were statistically significant, and if the PBM of the top-ranked candidate was markedly superior to that of the next-ranked candidate. Experimental peptide masses were assessed for systematic divergence from hypothetical calculated peptide masses, wherein random mass deviations were used to reject candidate identifications. Numerical simulation Our model of proteasome assembly was represented as a system of ordinary differential equations (ODEs). We numerically integrated these ODEs using the CVODE library in the SUNDIALS package [54] . A description of the model itself, along with the full set ODEs, can be found in the Supplementary Notes 1 and 2 . The concentrations of the different proteins in this model were estimated from experimental measurements in yeast [55] , and the interaction parameters (association rates, dissociation rates, affinities and so on) were taken from biolayer interferometry measurements ( Supplementary Fig. 2a ). How to cite this article: Wani, P. S. et al. Maturation of the proteasome core particle induces an affinity switch that controls regulatory particle association. Nat. Commun. 6:6384 doi: 10.1038/ncomms7384 (2015).